Few-femtosecond time-resolved measurements of X-ray free-electron lasers X-ray free-electron lasers, with pulse durations ranging from a few to several hundred femtoseconds, are uniquely suited for studying atomic, molecular, chemical and biological systems. Characterizing the temporal profiles of these femtosecond X-ray pulses that vary from shot to shot is not only challenging but also important for data interpretation. Here we report the time-resolved measurements of X-ray free-electron lasers by using an X-band radiofrequency transverse deflector at the Linac Coherent Light Source. We demonstrate this method to be a simple, non-invasive technique with a large dynamic range for single-shot electron and X-ray temporal characterization. A resolution of less than 1 fs root mean square has been achieved for soft X-ray pulses. The lasing evolution along the undulator has been studied with the electron trapping being observed as the X-ray peak power approaches 100 GW. Over the past several years, great progress has been made in the realization of high power X-ray free-electron lasers (FELs) [1] , [2] , [3] , [4] . The typical pulse duration from these sources can vary from several hundred femtoseconds down to a few femtoseconds with about 10 11 –10 13 photons per pulse. Such intense X-ray pulses, which are about 2–3 orders shorter and 8–10 orders brighter than pulses from storage ring-based third-generation light sources [5] , provide a revolutionary tool for ultrafast time-resolved X-ray studies with atomic spatial resolution. However, tremendous challenges remain in diagnosing such X-ray pulses with femtosecond temporal resolution. Conventional photodetectors do not have a fast enough response time in the few-femtosecond regime, while time-frequency correlation techniques widely used in the optical regime are also very difficult to realize because of the small cross-sections in nonlinear processes at X-ray wavelengths [6] . At X-ray FELs such as the Linac Coherent Light Source (LCLS) [2] , the X-ray pulse duration is typically estimated from the measured electron bunch duration [7] , [8] , [9] , [10] . While this is very helpful to set-up the machine for user experiments, the X-ray pulse duration could differ as much as a factor of two from that of the electron bunch, as reported by some early experiments (see, for example, refs 11 , 12 ). This could be due to non-uniform lasing inside the electron bunch since the intensity of the FEL power profile is strongly determined by time-dependent electron beam properties, such as the beam current, emittance and energy spread. Moreover, the jitter in beam current and energy also makes the pulse intensity and temporal profile fluctuate from shot to shot. All these factors can cause the X-ray pulse duration and temporal profile to deviate from that of the electron bunch. For proper interpretation of the photon experimental data, temporal characterization of the X-ray pulses on a shot-by-shot basis is critical and highly desired. For example, all nonlinear X-ray sciences utilizing X-ray FELs require a measure of the intensity, that is, photons per unit area per unit time. In the early experiments at LCLS [11] , [13] , the experimenters inferred the X-ray pulse duration to explain their results owing to lack of X-ray diagnostics. In the field of molecular imaging and nanocrystallography, ultrashort and temporally well-defined X-ray pulses are crucial as the radiation damage is expected and observed experimentally [14] , [15] . To overcome the challenges in femtosecond X-ray diagnostics, several techniques have recently been developed [16] . One of them is the terahertz streaking technique [17] , [18] , where a terahertz field is used to streak photoelectrons created from ionizing a noble gas with the X-ray pulse. By measuring the streaked photoelectron energy spectrum, the X-ray pulse temporal structure can be retrieved. This is a single-shot method with a best resolution reported to date of about 10 fs (refs 17 , 18 ). Multi-shot methods such as those based on spectral analysis [19] , [20] or correlation techniques [12] , [21] , [22] , [23] , [24] have also been explored; these typically yield the pulse duration but not the temporal distribution. We previously proposed characterizing the X-ray temporal structure by measuring the FEL-induced lasing effects on the electron beam [25] . A radiofrequency (rf) transverse deflector is adopted in conjunction with an electron beam energy spectrometer to measure the electron beam longitudinal (time-energy) phase space downstream of the FEL undulator. Since the lasing process in an FEL induces both electron energy loss and energy spread growth, the output electron longitudinal phase space will include a ‘footprint’ left by the emitted X-rays. Enabled by well-developed rf technology, this diagnostic method is simple, single shot and non-invasive to FEL operation. Furthermore, it covers a wide dynamic range and works for both soft and hard X-ray energies without requiring any configuration change. Here we report the X-ray temporal profile measurement at the LCLS with the recently commissioned X-band rf deflector system. We have achieved a temporal resolution of less than 1 fs root mean square (r.m.s.) in the soft X-ray regime (~1 keV) and ~4 fs r.m.s. in the hard X-ray regime (~10 keV). Since we actually measure the longitudinal phase space of the electron beam for X-ray pulse reconstruction, this reported diagnostic technique provides an ideal tool for studying the FEL lasing evolution and performance optimization. Electron trapping in the X-ray FELs has been observed as the pulse peak power approaches ~100 GW. X-ray temporal diagnostics using a transverse deflector A travelling wave, rf deflecting structure can provide high-frequency, time-varying transversely deflecting fields. The invention is nearly 50 years old [26] . It was adopted for low-energy electron bunch temporal measurements and lasing studies at Los Alamos infrared FEL in the 1980s (ref. 27 ), and recently this diagnostic device has been proposed for X-ray FEL facilities [28] , [29] . The action of the deflecting system on the electron bunch is analogous to a streak camera. The time variation of the transverse fields is used to create a temporal-spatial correlation in the electron bunch phase space. The resulting image on a downstream screen forms a ‘streak’ of the electron bunch, from which the pulse duration and temporal profile can be obtained. If this deflector streaks the electron beam horizontally and a dipole magnet disperses the beam vertically, we can obtain the full time-energy longitudinal phase space of the electron beam on a single shot by measuring the downstream transverse images [30] , [31] . At the LCLS, the existing S-band rf (2.856 GHz) transverse deflector provides a temporal resolution of about 10 fs r.m.s. at 5 GeV beam energy [7] . This resolution is determined by the deflector frequency, voltage and the electron beam properties. Such an S-band deflector is insufficient to resolve the bunch structure at full LCLS beam energy (~15 GeV). To achieve a better resolution, a transverse deflector working at an X-band frequency (11.424 GHz) was considered for the LCLS [32] , [33] with the deflecting structures and power couplers developed in the years that followed [34] , [35] . Since this frequency is a factor of four higher than the existing LCLS S-band deflecting structures thus allowing higher rf fields, it produces a faster, stronger transverse sweep of the beam, improving the temporal resolution over previous deflector designs. In the FEL process, when electrons wiggle in the undulator, the interaction between the electron beam and the radiation fields leads to a coherent energy modulation for electrons whose energy is near the FEL resonance with the fundamental radiation wavelength. This energy modulation develops into a density modulation (the so-called ‘microbunching’) along the undulator, itself inducing coherent radiation emission and even greater energy modulation. This collective interaction leads to a net energy transfer from electrons to photons. As a result, amplification of the radiation is achieved, while at the same time inducing electron energy loss and growth of the energy spread. This produces the ‘footprint’ that the FEL lasing process leaves on the electron beam’s longitudinal phase space. We extended the transverse deflector diagnostic scheme to retrieve the detailed X-ray pulse duration and temporal profile by measuring this lasing footprint [25] . The sketch in Fig. 1 shows the implementation of the deflecting system at the LCLS. Two 1-m-long X-band rf deflecting structures powered by one 50-MW klystron provide a 45-MeV c −1 nominal time-dependent horizontal kick to the beam [36] . The pre-existing, vertical-bend dipole magnet is used to measure the electron energy spectrum. A camera monitors the downstream cerium-doped yttrium aluminium garnet (Ce:YAG) crystal screen, capturing the transverse beam image. In this arrangement, the horizontal dimension of the measured image represents time while the vertical dimension represents energy. The horizontal scale of the image can be calibrated in absolute units of time by measuring the beam centroid position as a function of rf phase in degrees of X-band at the deflector (see Supplementary Fig. 1 ). Similarly, the vertical scale is calibrated with known beam energy shifts. The expected temporal resolution is about 1–3 fs r.m.s. depending on the beam energy [37] . Details about calibration and resolution can be found in the Supplementary Note 1 . 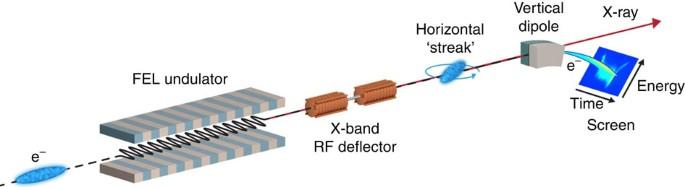Figure 1: Diagnostic layout of the X-ray temporal measurement. It includes the transverse deflector, the magnetic spectrometer and the Ce:YAG screen located downstream of the FEL undulator. Two 1-m-long X-band rf deflecting structures provide horizontal streaking followed by a vertical-bend dipole magnet for measuring the energy spectrum. A camera captures the transverse images of the electron beam density distribution on the diagnostic screen. Figure 1: Diagnostic layout of the X-ray temporal measurement. It includes the transverse deflector, the magnetic spectrometer and the Ce:YAG screen located downstream of the FEL undulator. Two 1-m-long X-band rf deflecting structures provide horizontal streaking followed by a vertical-bend dipole magnet for measuring the energy spectrum. A camera captures the transverse images of the electron beam density distribution on the diagnostic screen. Full size image Temporal profile reconstruction of soft X-ray pulses We use a soft X-ray example to demonstrate the procedure of measurement and temporal reconstruction. The electron beam energy is 4.7 GeV with FEL operating at a resonant photon energy of 1.0 keV. We first suppressed the lasing process by perturbing the electron horizontal trajectory at the beginning of the undulator and then recorded hundreds of what we refer to as ‘lasing-off’ or ‘baseline’ longitudinal phase space images on the screen. 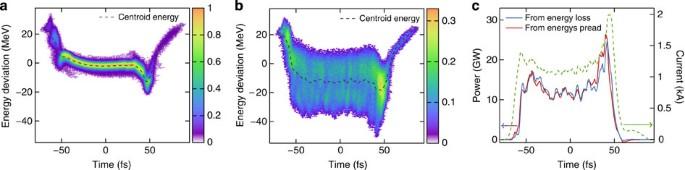Figure 2: Temporal profile reconstruction. The electron bunch charge is 150 pC with an energy of 4.7 GeV to produce photons at 1.0 keV. The measured single-shot longitudinal phase space images are shown ina: ‘lasing off’ andb: ‘lasing on’. Comparing the ‘lasing-off’ with the ‘lasing-on’ images, we reconstruct the X-ray power profile as shown incfrom the time-dependent energy loss (blue curve) and energy spread growth (red curve). The electron current profile (green-dashed line) is also shown inc. The example shown here is measured just after saturation with a total X-ray pulse energy of 1.5 mJ. The bunch head is to the left in these plots and throughout. Figure 2a shows a typical single-shot baseline image. Its projection onto time gives the electron bunch current profile. Next, we restored the electron trajectory and recorded the ‘lasing-on’ images for normal operation (a single shot is shown in panel b). On comparing panel b with a in Fig. 2 , one can clearly see the time-resolved energy loss and energy spread growth due to the lasing process. Figure 2: Temporal profile reconstruction. The electron bunch charge is 150 pC with an energy of 4.7 GeV to produce photons at 1.0 keV. The measured single-shot longitudinal phase space images are shown in a : ‘lasing off’ and b : ‘lasing on’. Comparing the ‘lasing-off’ with the ‘lasing-on’ images, we reconstruct the X-ray power profile as shown in c from the time-dependent energy loss (blue curve) and energy spread growth (red curve). The electron current profile (green-dashed line) is also shown in c . The example shown here is measured just after saturation with a total X-ray pulse energy of 1.5 mJ. The bunch head is to the left in these plots and throughout. Full size image To reconstruct the time-dependent X-ray power profile from the energy loss, we first ‘slice’ the beam image along the time dimension to get the time-dependent beam parameters such as the centroid energy E ( t i ) and current I ( t i ) in each time slice t i . By comparing the lasing-on and lasing-off sliced data, we can obtain the time-resolved mean energy loss Δ E ( t i ), from which the absolute power can be determined directly as P ( t i )=Δ E ( t i ) × I ( t i )/ e (ref. 25 ). The slight slippage of the radiation pulse relative to the electron bunch is neglected here, as it is typically a small fraction of the achieved temporal resolution. The reconstruction is done shot by shot and the incoming electron energy jitter has to be subtracted to determine the absolute power. In a simple way, the absolute power scale of the reconstructed X-ray profile can also be calibrated against the total X-ray pulse energy, as measured simultaneously at a calibrated gas detector [38] . In this way, the electron beam energy jitter issue can be ignored during data processing. A similar, alternative technique based on an extension of the analysis in ref. 39 utilizes the change in energy spread to retrieve the X-ray power profile. This can be written as , where the and are the time-dependent energy spread with lasing on and off, respectively. In this proportional form, the method requires an independent measurement of the pulse energy from the gas detector for absolute power normalization. These two methods, using the time-resolved energy loss or energy spread change, generally agree very well before or near FEL power saturation, as shown in Fig. 2c . Details about the reconstruction procedure are further discussed in Supplementary Note 2 and Supplementary Fig. 2 . It should be noted that with stable machine conditions the lasing-off images need only to be sampled once, while lasing-on images can be subsequently recorded during normal FEL operation, thus permitting continuous, single-shot, time-resolved X-ray pulse measurements. With an electron bunch charge of 150 pC, the achievable X-ray pulse duration is about 50–150 fs full-width at half-maximum (FWHM) as shown in Fig. 2c , depending on how much the electron bunch is compressed upstream. Even shorter X-ray pulses are desired for some scientific experiments such as biomolecular imaging [14] and time-resolved pump-probe spectroscopy in femtochemistry [40] . At the LCLS, two experimental methods—a low-charge (20 pC) mode [41] and a slotted-foil emittance spoiling scheme [42] —have been successfully developed to produce sub-10 fs X-ray pulses. However, until now, there has been no diagnostics reported that can measure the X-ray pulses at a resolution of a few femtoseconds or better. Using this reported X-band rf deflector, we are able to characterize the electron bunch and the X-ray pulse with femtosecond resolution. 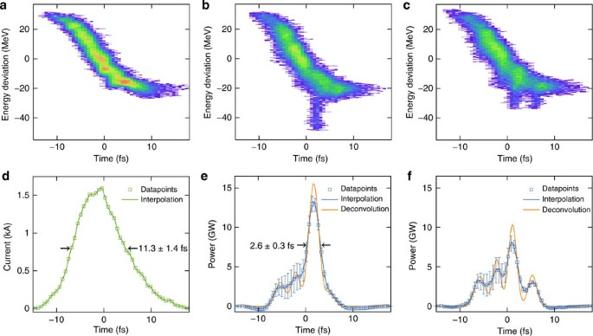Figure 3: Measurements of sub-10 fs X-ray pulses. The electron bunch charge is 20 pC with electron beam energy of 4.7 GeV. (a) One single-shot lasing-off image; (b,c) two single-shot lasing-on images; (d) the current profile showing a bunch duration of ~11 fs full-width half maximum (FWHM). The reconstructed X-ray temporal profiles from the measured slice energy loss are shown ineandf. X-ray pulse duration of less than 3 fs FWHM is measured ine. The data points represent the measured beam parameters at the discrete time slices, where the errors are derived from the averaging of multiple baseline images, and the deconvolution has been applied using the measured time resolution. Figure 3 shows measurements of a 20-pC bunch with the FEL configured for an X-ray photon energy of 1.0 keV. With this overcompression operation mode (see panel a) the electron bunch duration is measured to be ~11 fs FWHM with an experimentally determined resolution of 0.8±0.1 fs r.m.s. The two examples of lasing-on shots in panels b and c show that it is mainly the high-current core of the beam that contributes to lasing. By comparing the lasing-on (b,c) images with the lasing-off (a) one, the X-ray power profiles are reconstructed in e and f (blue curves). Finally, temporal profiles with applied deconvolution using the measured time resolution are presented as well. In panel e, the pulse duration is 2.6±0.3 fs FWHM that approaches the expected value for a single, coherent self-amplified spontaneous emission spike at ~1 keV. Another single shot, shown in f, clearly reveals multiple spikes with similar widths. Further discussions about deconvolution can be found in Supplementary Note 3 and Supplementary Fig. 3 . Figure 3: Measurements of sub-10 fs X-ray pulses. The electron bunch charge is 20 pC with electron beam energy of 4.7 GeV. ( a ) One single-shot lasing-off image; ( b , c ) two single-shot lasing-on images; ( d ) the current profile showing a bunch duration of ~11 fs full-width half maximum (FWHM). The reconstructed X-ray temporal profiles from the measured slice energy loss are shown in e and f . X-ray pulse duration of less than 3 fs FWHM is measured in e . The data points represent the measured beam parameters at the discrete time slices, where the errors are derived from the averaging of multiple baseline images, and the deconvolution has been applied using the measured time resolution. Full size image Lasing evolution of hard X-ray FELs With this diagnostic tool established, we can study the FEL lasing process and more effectively improve the accelerator and FEL performance. For example, in the hard X-ray regime, coherent diffraction imaging of complex molecules requires a large number of photons (for example, ~10 13 photons in ~10 fs pulse) that correspond to terawatt peak power [43] , [44] . This requirement is at least one order of magnitude higher than achievable at existing FEL facilities. Tapering the undulator strength after FEL saturation is a well-known method for achieving higher FEL power (see, for example, refs 45 , 46 , 47 ). The FEL resonant wavelength is , where λ u is the undulator period, K is the normalized undulator strength parameter and γ is the electron energy in units of the rest energy mc 2 . In the tapered section, the undulator strength ( K value) is properly matched to the FEL-induced energy loss of the electron beam, allowing some electrons to be continuously trapped within a longitudinal phase space separatrix, or ‘FEL radiation bucket’ [45] . In this way we expect to extract additional radiation power after the saturation of the FEL. As an example, we have measured the evolution of FEL lasing along the undulator at a photon energy of 10.2 keV (see Fig. 4 ). During these measurements we suppress the lasing over a section of the undulator by perturbing the electron trajectory with steering coils (kickers) located along the undulator [48] . The trajectory is nominal for lasing up to the applied kicker, so the reconstructed X-ray power profile represents the lasing performance at that point. A taper varying quadratically along the undulator distance was applied beyond the 21st undulator segment (U21; each segment is 3.4 m long) and optimized to achieve the maximum pulse energy at the end of the undulator beamline at U33. The X-ray pulse energy is increased from ~1 mJ at U25 to ~2.8 mJ at U33. This indicates that the post-saturation taper improves the photon pulse energy by more than a factor 2, as also reported earlier [48] . Here from the longitudinal phase space measurements, we clearly observe an energy gap in the deep-saturation regime, which means some electrons have been trapped and continuously decelerated with this optimized taper set-up. To understand the trapping effect, the electron resonant energy along the undulator distance is derived from the tapered undulator K value using the FEL resonance condition, as plotted with red-dashed lines on the phase space images in panel a. It shows that the mean energy of the trapped electrons is consistent with the FEL resonant energy in the taper regime, which makes it possible to extract additional photons after FEL saturation. If there is no post-saturation taper applied, the measured longitudinal phase space at U33 is similar to the one at U25, and the pulse energy stays at 1 mJ level. In this way the reported new diagnostic technique provides an effective tool for taper optimization in FELs. 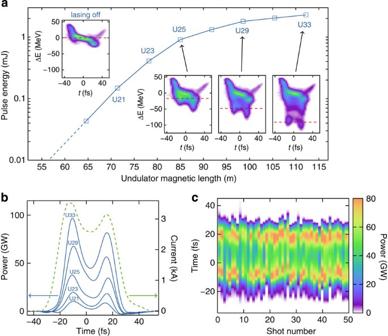Figure 4: Lasing evolution of hard X-ray free electron lasers. The electron bunch charge is 150 pC with beam energy of 15.2 GeV, and the photon energy is 10.2 keV. (a) The measured electron beam longitudinal phase space distribution at different undulator positions. The blue line with squares shows the measured FEL power gain curve. We show sample lasing-on images at U25, U29, and U33 and lasing-off images, where the red-dashed lines on the images indicates the resonant electron energy according to the undulatorKvalues used. In the deep saturation point at U33, trapped electrons are evident. (b) The X-ray power profiles ranging from pre-saturation to deep saturation are shown at U21, U23, U25, U29 and U33, and the electron current profile is also included with green-dashed line. (c) The power profiles from 50 consecutive shots after U33 are plotted, where we illustrate the pulse shape stability with centre-of-mass correction. Figure 4: Lasing evolution of hard X-ray free electron lasers. The electron bunch charge is 150 pC with beam energy of 15.2 GeV, and the photon energy is 10.2 keV. ( a ) The measured electron beam longitudinal phase space distribution at different undulator positions. The blue line with squares shows the measured FEL power gain curve. We show sample lasing-on images at U25, U29, and U33 and lasing-off images, where the red-dashed lines on the images indicates the resonant electron energy according to the undulator K values used. In the deep saturation point at U33, trapped electrons are evident. ( b ) The X-ray power profiles ranging from pre-saturation to deep saturation are shown at U21, U23, U25, U29 and U33, and the electron current profile is also included with green-dashed line. ( c ) The power profiles from 50 consecutive shots after U33 are plotted, where we illustrate the pulse shape stability with centre-of-mass correction. Full size image The evolution of the X-ray power profile along the undulator is demonstrated in Fig. 4b . The X-ray power profile possesses a double-horn temporal structure similar to the electron bunch current. At the end of the undulator, the peak power is approaching 100 GW. From 50 consecutive shots of the measured X-ray power profiles at U33 (see panel c), we can see the pulse duration is relatively stable with a double-horn temporal structure consistently observed. In this deep saturation example, the total radiation slippage relative to the electron bunch is estimated to be less than 0.5 fs and is negligible compared with the resolution limit. Single-shot measurements of the electron and X-ray temporal profiles have been carried out at the LCLS using the recently commissioned X-band rf transverse deflector. This provides an excellent X-ray temporal diagnostic tool largely independent of photon energy, together with a large dynamic range. The data processing for reconstruction of the X-ray temporal profiles is simple and reliable, and can provide a constant stream of non-invasive, single-shot X-ray temporal profiles during user experiments. The measured resolution is below 1 fs r.m.s. at soft X-ray energies and ~4 fs r.m.s. at hard X-ray energies. A pulse duration of less than 3 fs FWHM at soft X-ray energy has been measured, and the electron trapping in X-ray FELs was experimentally observed in the deep-saturation regime. To further improve the temporal resolution, one can increase the deflecting strength by either adding more deflectors or upgrading the existing power source with rf pulse compression technology [49] , [50] , [51] . It is also possible to further optimize the electron beam optics by adding quadrupole magnets. Improvements like these would allow us to approach sub-femtosecond resolution at hard X-ray energies. Experiment set-up The longitudinal electron bunch phase space distributions have been measured using a scintillation screen made of Ce:YAG. This Ce:YAG screen has a diameter of 1.5-inch and a thickness of 50 μm; it is tilted by 5° with respect to the electron beam axis. Such a relatively large screen is chosen to accommodate the beam position jitter mainly caused by the beam arrival time and rf phase jitter. The screen is finally imaged by a charge-coupled device (CCD) camera equipped with standard optics and viewed via an upstream mirror-like foil rotated by 25°. The 5° tilt angle steers the coherently emitted optical transition radiation by the upstream foil into the direction of specular reflection away from the CCD camera. The CCD chip of the camera has a bit depth of 12 bits and consists of 1,394 × 1,040 pixels with 4.65 × 4.65 μm 2 pixel size. The magnification provided by a 55-mm telecentric lens is 1:6.4, leading to an apparent pixel size of 29.8 × 29.8 μm 2 . The read-out frame rate of the CCD camera was 10 Hz for the data recorded in this paper, but an upgrade to a camera capable of operating at the full LCLS repetition rate of 120 Hz has been ready since the beginning of 2014. The CCD images have been post-processed before the final analysis using standard image processing tools to remove noise. Error analysis The main errors in the presented measurements are governed by statistical errors in the multi-shot calibrations, which are dominated by beam position jitter at the Ce:YAG screen. The final measurement errors, for example, of the pulse duration or time resolution, have been calculated by applying error propagation rules. Systematic errors due to initial electron beam phase space correlations have been identified and corrected. Further details on errors can be found in the Supplementary Note 1 . How to cite this article : Behrens, C. et al. Few-femtosecond time-resolved measurements of X-ray free-electron lasers. Nat. Commun. 5:3762 doi: 10.1038/ncomms4762 (2014).